Frequent cases of RAS-mutated Down syndrome acute lymphoblastic leukaemia lackJAK2mutations Children with Down syndrome (DS) and acute lymphoblastic leukaemia (ALL) have poorer survival and more relapses than non-DS children with ALL, highlighting an urgent need for deeper mechanistic understanding of DS–ALL. Here, using full-exome or cancer genes-targeted sequencing of 42 ALL samples from 39 DS patients, we uncover driver mutations in RAS, (KRAS and NRAS) recurring to a similar extent (15/42) as JAK2 (12/42) mutations or P2RY8-CRLF2 fusions (14/42). RAS mutations are almost completely mutually exclusive with JAK2 mutations ( P =0.016), driving a combined total of two-thirds of analysed cases. Clonal architecture analysis reveals that both RAS and JAK2 drove sub-clonal expansions primarily initiated by CRLF2 rearrangements, and/or mutations in chromatin remodellers and lymphocyte differentiation factors. Remarkably, in 2/3 relapsed cases, there is a switch from a primary JAK2- or PTPN11-mutated sub-clone to a RAS-mutated sub-clone in relapse. These results provide important new insights informing the patient stratification strategies for targeted therapeutic approaches for DS–ALL. Acute lymphoblastic leukaemia (ALL) is the commonest cancer-related cause of death in children and young adults, and the most common malignancy of paediatric age [1] , [2] . Children with Down syndrome (DS) have an approximately 10–50-fold higher incidence of leukaemias than children without DS (non-DS), including B-cell progenitor cell ALL (BCP–ALL) and most types of acute myeloid leukaemia (AML) [3] , [4] , [5] , with myeloid leukaemia of DS (ML–DS) being recognized as a DS-specific disease [6] . In addition to a constitutional trisomy 21, DS leukaemias show a distinct pattern of acquired genetic changes. Almost all cases of ML–DS are characterized by in utero -acquired typical mutations in the transcription factor GATA1 (refs 7 , 8 , 9 ), and DS–ALL shows increased incidence of mutations in the tyrosine kinase janus kinase 2 ( JAK2 ) [10] , [11] , [12] , and greater abundance of rearrangements/mutations at the cytokine receptor-like factor 2 ( CRLF2 ) locus [11] , [13] than non-DS–ALL. Next generation sequencing (NGS) is opening new insights into the mechanisms of leukaemogenesis and detecting the spectrum of therapeutic targets [14] . Exome and genome sequencing studies of childhood acute leukaemias revealed partially overlapping profiles of driver mutations underlying the unique nature of each leukaemic type. Acute megakaryoblastic leukaemia (AMKL) in children with DS were shown to harbour secondary driver mutations in genes of the cohesion complex, epigenetic regulators and signalling pathways which reveals the similarity with the driver mutational profiles in non-DS–AML [15] , [16] , [17] , [18] , [19] , [20] , [21] . Given that constitutional trisomy 21 in DS highly predisposes children to most types of leukaemia, and to a characteristic set of mutations that set them apart from non-DS leukaemias (GATA1, CRLF2, JAK2), it remains unclear whether the spectra of driver mutations in DS–ALL would be more similar to ML–DS or to non-DS–ALL. The DS–ALL patients have much worse event-free and overall survival rates than non-DS–ALL [14] . Leukaemic blasts from ML–DS are far more sensitive to chemotherapeutic agents than cells from non-DS–AML, but blasts from DS–ALL do not differ in this sensitivity to non-DS–ALL blasts [22] . Therefore, while in ML–DS, the reduced dose chemotherapy has been successfully applied to reduce treatment-related mortality, this strategy is not recommended for DS–ALL, (apart from only for a small minority of low-risk DS–ALLs [14] ). This fact is further corroborated by the largest study of its kind on 653 DS–ALL patients, which has shown that poorer survival rates in DS–ALL are only partially due to higher treatment-related mortality, and are predominantly due to a much higher incidence of relapse than in non-DS–ALL children [14] . The worse outcome could partly be explained by the absence (or very rare appearance) of the favourable prognosis-associated genetic lesions in DS (hyperdiploidy and ETV6-RUNX1 fusions) [23] . All this demonstrates an urgent need for further DS–ALL patient sub-stratification, analysis of the full spectrum of acquired mutations and a deeper understanding of the mechanisms by which they contribute to the evolution of the primary and relapsing leukaemia. Here we report the detailed driver mutational profiles of 42 ALL samples from 39 DS patients by full-exome or cancer genes-targeted sequencing. In three patients, the spectra of driver mutations are compared between the samples at primary diagnosis and the relapse. We discover driver mutations in RAS (KRAS and NRAS) recurring to a similar (or higher) extent (15/42) as JAK2 (12/42) mutations, or P2RY8-CRLF2 fusions (14/42). Interestingly, driver mutations in RAS pathway are mutually excluding with JAK2 mutations, P =0.016, and cumulatively (JAK2 and RAS combined) were detected in 66% of DS–BCP–ALL primary leukaemias and relapses. Clonal architecture ( n =20/27 cases) and clonal evolution in relapse ( n =3 cases) have shown that both JAK2 and RAS mutations are likely sub-clonal expansions, not initiating events. The dominating events are a combination of CRLF2 rearrangements, mutations in epigenetic (chromatin) modifiers, classical tumour suppressors and/or lymphocyte differentiation factors, and these are cumulatively present in 93% of cases with no significant association with either JAK2 or RAS sub-groups. Overall, our data suggest that therapeutic outcomes for DS–ALL could be improved by a personalized approach to driver mutation profiled cases, with inclusion of RAS (particularly KRAS) inhibitors and/or chromatin modifier enzyme inhibitors to the current therapeutic strategies. Here we report the detailed analysis of the mutational profiles of 42 DS–ALL samples from 39 individuals. Of these, 16 patients with tumour at diagnosis (T1) and remission samples were analysed by exome sequencing, and the other 23 patients with tumour sample at diagnosis were analysed by targeted sequencing of coding exons of 387 cancer-related genes ( Supplementary Data 1, and Methods ). For three patients, additionally to tumour at diagnosis, relapsed tumour sample (T2) was sequenced. In addition, all samples were analysed by direct genomic DNA end-point PCR for the presence of the P2RY8-CRLF2 fusion events ( Supplementary Fig. 1 ). This event represents the most frequent cause of CRLF2 rearrangement in DS–ALL [14] . All studied DS–ALLs, with exception of one T-cell leukaemia (very rare in DS) had the BCP–ALL mostly of cALL (B-II) or pre-B (B-III) sub-types. Mutation rates in DS–ALL were on average 0.2 mut per Mb with C>T mutations comprising 60% of all mutations ( Supplementary Data 2 ). In Fig. 1 , we summarized all point mutations, somatic copy number aberrations and P2RY8-CRLF2 fusion events that pass the criteria for putative driver events (Methods). Out of 42 leukaemia samples, (belonging to 39 individuals), only one sample showed no obvious putative driver mutations. The other 41 samples have shown mutations in one or more of driver genes grouped into functional families: the JAK–STAT pathway (JAK2, IL7R), the RAS/receptor tyrosine kinase (RTK) pathway (KRAS, NRAS, PTPN11, NF1, FLT3, KIT), Cohesin complex (SMC3), epigenetic modifiers/remodellers of DNA (DNMT3A) or chromatin (NCOR1, BCOR, ASXL1, HDAC9, SETD2, EZH2, SUZ12, CREBBP, EP300), classical tumour suppressor genes (CDKN2A, TP53, APC) or lymphoid differentiation factors/markers (IKZF1, ETV6, NOTCH1, VPREB1). 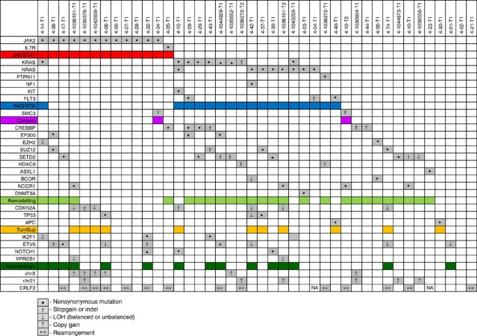Figure 1: Somatic mutations and CNAs in DS–ALLs. Each column represents a tumour sample. Each line represents a cancer gene or a pathway. Grey cells with a symbol represent a somatic event in the corresponding gene. Coloured cells represent all cases with a somatic event in a pathway. Figure 1: Somatic mutations and CNAs in DS–ALLs. Each column represents a tumour sample. Each line represents a cancer gene or a pathway. Grey cells with a symbol represent a somatic event in the corresponding gene. Coloured cells represent all cases with a somatic event in a pathway. Full size image RAS mutations are as recurrent as JAK2 mutations in DS–ALL RAS genes of the RAS–RTK pathway harboured putative driver mutations in 36% of BCP–ALLs cases uncovering KRAS (9/41) and NRAS (8/41) genes as one of the most important acquired genetic effectors in DS–ALL. Altogether, 66% of BCP–ALL tumours had driver mutations in either RAS or JAK2 genes. RAS mutations totally mutually exclude JAK2 in DS leukaemia Mutations in JAK2 on one hand and RAS on the other hand were statistically significantly mutually exclusive ( P =0.016 using Fisher’s exact one-sided test). Only one sample (4–14-T1) had mutations in both JAK2 and KRAS. Detailed analysis of the clonal architecture of this sample ( Fig. 2 ), revealed that JAK2 mutation was present in 80% of cells (nearly 100% of blasts), whereas mutations in KRAS and losses of EZH2 and IKZF1 were all present with a frequency of around 45%. These observations could be explained by co-existence of a founder clone with JAK2 mutation alone and one or more sub-clones with JAK2, KRAS, EZH2 and/or IKZF1 mutations. Potential co-existence of mutations in JAK2 and KRAS genes in the same leukaemic cells was observed only in this one sub-clone from all cases in the entire study. Existence of multiple sub-clones in 4–14-T1 was also suggested through immunophenotypic examination where two morphologically different kinds of blasts were identified. This was also the only case in the study that had the immature (pre-pre-B or B-I; that is, CD10-) immunophenotypic diagnosis in a fraction of blasts, and the common (cALL or B-II) diagnosis for the other fraction of blasts. 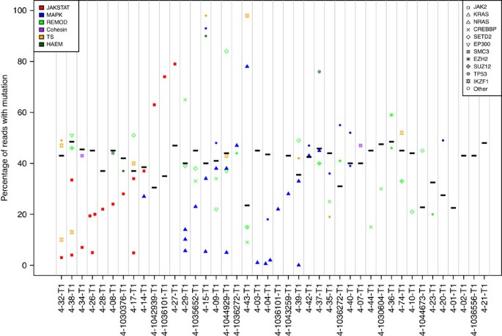Figure 2: Clonal architecture analysis. Percentage of reads from high-throughput sequencing (HTS) supporting the somatic mutations in 42 studied DS–ALL samples. Colours represent different pathways. Symbols represent different driver genes. Horizontal bars represent half of fraction of blasts in the tumour sample. Figure 2: Clonal architecture analysis. Percentage of reads from high-throughput sequencing (HTS) supporting the somatic mutations in 42 studied DS–ALL samples. Colours represent different pathways. Symbols represent different driver genes. Horizontal bars represent half of fraction of blasts in the tumour sample. Full size image Both RAS and JAK2 are sub-clonal driver events in DS-ALL In total, 74% of the RAS- and JAK2-mutated cases (20/27) also contained other mutations in different gene families. Clonal architecture analysis ( Fig. 2 ) has shown that in almost all cases, these other gene family mutations substantially outnumbered the percentage of cells bearing the RAS or JAK2 genes mutations. For example, in the tumour 4–29-T1, KRAS mutations (6.2–16.6% of reads) in all likelihood were secondary to the mutations in chromatin remodelling genes (CREBBP: 65% of reads, SETD2: 46 and 39% of reads). Strikingly, 11 RAS- or JAK2-driven sub-clones had low-variant allele frequencies between 1 and 10% further underlining their secondary origin. Moreover, in nine tumours, two or three RAS or JAK2 driver mutations were detected. We also report that in five cases, where such mutations (4–04-T1:NRAS; 4–29-T1:KRAS (three mutations); 4–38-T1:JAK2; 4–26-T1:JAK2) were located close to each other (<100 bp), none of them were found on the same sequence reads (same allele) suggesting that they drive different sub-clones in the tumour ( Fig. 2 ; Supplementary Data 3 and 4 ). Gains of extra copies of chromosome 21 (six cases, Supplementary Fig. 2 ) in most cases (and in both exome-sequenced relapse cases) as well as RAS or JAK2 mutations were observed in the sub-clones. In the three relapse cases analysed ( Fig. 3 ), the dominant changes present in both primary tumour and the relapse were neither JAK2 nor RAS mutations, but mutations in classical tumour suppressor genes (CDKN2A), B-lymphocyte differentiation factors (VPREB1), chromatin remodeller family genes (HDAC9, NCOR1) and/or a P2RY8-CRLF2 fusion, indicating that these were most likely the initiating events. The putative driver events in genes of these gene families were detected cumulatively in 93% of cases, with no significant association with either JAK or RAS groups. The data are compatible with the evolutionary chain of events in which these events initiate the clonal expansion, followed by a subsequent formation of mutually excluding JAK2- or RAS-mutated sub-clones that ‘explode’ the sub-clonal proliferation. 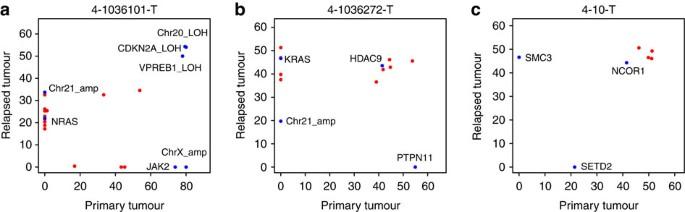Figure 3: Comparison of the somatic mutations between the primary leukaemias and relapses. Pairwise comparisons of percentages of reads with the mutations and somatic copy number aberrations (SCNAs) between primary leukaemias and relapse samples for: 4-1036101 (a), 4-1036272 (b), 4–10 (c). Red dots are passenger mutations, and blue dots are the driver mutations. NB: for 4–10 only 387 cancer genes were sequenced. NB: in patients 4-1036272 and 4–10 P2RY8-CRLF2 rearrangement was persistent in primary leukaemia and relapse, please seeSupplementary Fig. 1for an example. Figure 3: Comparison of the somatic mutations between the primary leukaemias and relapses. Pairwise comparisons of percentages of reads with the mutations and somatic copy number aberrations (SCNAs) between primary leukaemias and relapse samples for: 4-1036101 ( a ), 4-1036272 ( b ), 4–10 ( c ). Red dots are passenger mutations, and blue dots are the driver mutations. NB: for 4–10 only 387 cancer genes were sequenced. NB: in patients 4-1036272 and 4–10 P2RY8-CRLF2 rearrangement was persistent in primary leukaemia and relapse, please see Supplementary Fig. 1 for an example. Full size image Ras-driven sub-clones can replace other drivers in relapse In two cases where primary and relapsed tumours were available ( Fig. 3 , Supplementary Data 5 ), the primary leukaemia had mutations in the JAK–STAT family (JAK2 in patient 4-1036101) or PTPN11 (in patient 4-1036272) present in nearly all blast cells with no RAS–RTK family mutations. Notably, in both relapse cases the JAK–STAT- or PTPN11-mutated sub-clones completely disappeared after standard chemotherapy, and were replaced by NRAS- and KRAS-mutated sub-clones. Comparing DS-ALL driver profiles to other leukaemia types In order to investigate potential similarities between the repertoires of secondary and tertiary drivers of DS–ALL and other types of leukaemia, we performed a comparison of the prevalence of driver mutations by hierarchical clustering ( Supplementary Fig. 3 , Supplementary Data 6 ) of DS–ALL from this study ( n =42), with ML–DS ( n =57), five different types of non-DS–ALL (totalling 231 patients) and three different types of non-DS–AML (totalling 431 patients) that were analysed by NGS in recently published studies, (referenced in Supplementary Fig. 3 ). With this analysis, we also asked the question: to what extent the primary events that are hitherto known as specific characteristics of DS leukaemias (trisomy 21, CRLF2 and GATA1) determine the repertoire of further driver events? This is why in this analysis we excluded these dominant, DS-specific primary events and focussed on similarities/dissimilarities of the secondary, tertiary and further driver event profiles. Remarkably, the secondary/tertiary driver profiles of DS–ALL and ML–DS were more similar to each other, than to most other non-DS–ALL or AML types ( Supplementary Fig. 3 ), apart from non-DS near-diploid ALL and non-DS–AMKL. There were also subtle differences: genes of the epigenetic modifier gene family were mutated in 62% of DS–ALL, similar to the percentages found in hypodiploid non-DS–ALL [15] and slightly higher than in ML–DS. Individuals with DS have a paradoxical association with cancer, with a reduced incidence of most solid tumours, but an increased incidence of all types of leukaemia in childhood, due to mechanisms that are only partially understood [24] . The mechanistic paradigms currently explaining DS–ALL leukaemogenesis paint an incomplete picture: CRLF2 overexpression has been seen as the most frequently recurrent event, which then selects for events activating the JAK2 pathway in approximately a third of the CRLF2-rearranged cases [10] , [11] , [12] , [25] . In western populations, the frequency of CRLF2 rearrangements and/or overexpression ranges around 5–12% in non-DS–ALL and up to 62% in DS–ALL [11] , [13] , [26] . CRLF2 mutations alone don’t generate dominant relapse clones [26] . JAK2 mutations occur in a third of CRLF2-rearranged/overexpressed DS–ALL cases, and predispose to high risk and increased relapse incidence in non-DS–ALL [11] , [13] , [26] . In DS–ALL, neither CRLF2 rearrangements nor JAK2 mutations have a prognostic value [14] . The deeper understanding of the mechanisms of leukaemogenesis in DS–ALL remains an urgent need, especially the insights into the nature of molecular changes in relapsing cases, which are still the predominant reason for the poor survival rate in children with DS-ALL [14] . Our study leads to several new insights: (i) DS–ALL have a large proportion of driver mutations in KRAS and NRAS genes that are recurrent to a similar extent as JAK2 mutations or P2RY8-CRLF2 fusions, (ii) RAS mutations are almost completely mutually exclusive with JAK2 mutations down to the level of individual minor sub-clones. Remarkably, by retrospective analysis of the recently published exome-sequencing studies of ML-DS [16] , [18] , we uncovered the complete mutual exclusion of JAK–STAT and RAS–RTK family genes (co-occurrence in 0/28 cases) in ML–DS indicating a likely upstream point of sharp bifurcation between the activations of the two signalling pathways, regardless of the main leukaemia type, (iii) high-percentage representation in clonal architecture, as well as presence in both primary leukaemias and relapses indicate that the likely initiating oncogenic events in DS–ALL are mutations in chromatin remodellers, classic tumour suppressors, B-lymphocyte differentiation factors and/or CRLF2 rearrangements followed then by sub-clonal expansions of mutually excluding JAK- or RAS -mutated sub-clones. Our data support the scenario (depicted in Fig. 4 ) in which these events initiate DS–ALL. Sub-clones then accumulate mutually excluding mutations in either the JAK2 gene or the KRAS and NRAS genes. RAS mutations in many cases seem to appear in later sub-clones, or in relapses, accompanied by the complete disappearance of JAK2 mutations and a gain of extra copies of chr21, but all the while retaining the initiating events. 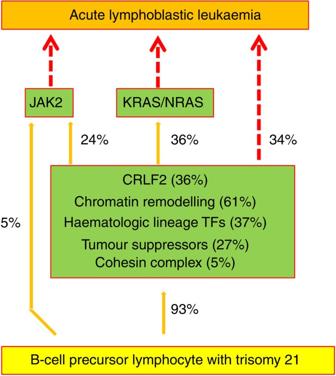Figure 4: Molecular multistep model of leukaemogeneis in DS–ALLs of BCP origin. Green boxes depict the pathways and gene families involved in tumorigenesis. Percents of tumours with mutations in indicated pathways are given in parentheses. Figure 4: Molecular multistep model of leukaemogeneis in DS–ALLs of BCP origin. Green boxes depict the pathways and gene families involved in tumorigenesis. Percents of tumours with mutations in indicated pathways are given in parentheses. Full size image Our findings on mutual exclusiveness of JAK2 and RAS mutations are concordant with the previous observations, where either JAK or RAS mutations were found dominating in different sub-types of childhood B-precursor ALL [27] . Our results put a particular spotlight on KRAS mutations, finding them in 21% of DS–ALL (compared with 0%, 2.9%, 9.1%, 18% and 20% respectively, in different cytogenetic sub-types of non-DS–ALL and AML [15] , [16] , [17] , [18] , [19] , [20] . In paediatric non-DS–ALL with an ETV6-RUNX1 translocation [21] , KRAS mutations were present in 10.5% of cases. KRAS mutations are also prevalent in many solid tissue tumours, and are associated with particularly poor prognosis [28] . In line with these data, we find that majority of KRAS-mutated primary DS–ALLs had poor outcome (death or relapse). The activated KRAS protein has also been proven as particularly difficult to counteract by pharmaceutical therapy, and was until recently deemed ‘un-druggable’ [29] . The recent development of deltarasin, a compound that disrupts the KRAS membrane association by blocking the farnesylated tail of KRAS binding to PDEδ [14] offers new hope for many KRAS-mutated cancers, and among them for probably the most progressive sub-clonal and relapsed expansions in DS–ALL. Our data suggest that standard chemotherapy managements for DS–ALL could be improved by patient stratification based on mutational profile, potentially considering a more aggressive and modified approach for a fraction of cases with RAS (in particular KRAS) mutations, suggesting the addition of KRAS inhibitors (deltarasin) and/or chromatin modifier enzyme inhibitors to therapeutic strategies. Patient samples Surplus clinical or archived clinical material was collected by the tissue bank of the Italian Association for Paediatric Haematology-Oncology. In accordance with the Declaration of Helsinki, informed written consent was obtained by the tissue bank for all subjects. Samples were processed and stored in the tissue bank at The Blizard Institute, which is licensed for tissue storage and monitored by UK-Human Tissue Authority. Detailed clinical description of studied DS–ALLs is provided in the Supplementary Data 1 . Detailed cytogenetics was available in 21 cases, and no hyperdiploid cases were detected. Only three cases had translocations: patient 4–29-T1 had a t(8;14)(p11.2;q32), patient 1036556 had a t(12:21), and the only patient with T-ALL (4–36-T1) had a t(7;11)(P22;Q23). Exome sequencing The overall methodology was as previously described [16] , [30] . DNA was extracted from the frozen samples using the QIAamp DNA Mini Kit (Qiagen), exome capture was performed using the SureSelect Human Exome v5 50 Mb (Agilent Technologies) kit and targeted capture of 387 cancer-related genes (1.6 Mb; Supplementary Data 7 ) was performed with SureSelect custom design protocol. In total, 387 cancer-related genes were selected based on mutational profiles in COSMIC v67 database taking into account fractions of truncating and recurrent mutations in different tumour types and include all Cancer Genes from recent reviews [31] , [32] . Sequencing was conducted on Illumina HiSeq2000 instrument with paired-end 105 nt reads. Burrows–Wheeler Aligner software was used to align the sequence reads to the human reference genome NCBI build (GRCh37/hg19). SAMtools was used to remove PCR duplicates and to call single-nucleotide variants. Detection of small insertions and deletions (smINDEL) was conducted with Pindel 0.2.2 software. The search for somatic mutations was restricted to the regions that were covered at least 20-fold. The average sequence coverage for the target region was 355 × ( Supplementary Data 8 ). Low-variant allele frequencies of oncogenic sites in JAK2 and RAS genes were examined to reveal minor tumour sub-clones. Average coverage of these sites across all samples was 409-fold. Low-variant allele frequencies mutations were selected if they met the following criteria: at least 2 reads on each strand and minimum 6 reads total, supporting the mutation) ( Supplementary Data 4 ). The full lists of coding somatic mutations were retrieved for tumours from the patients for which sample of blood in remission was available. Mutation was considered somatic if it was called in the tumour sample with quality score more than 50 and corresponding position in the constitutional DNA was covered more than 20-fold and was 100% represented by the reference allele ( Supplementary Data 2 ). In the tumours for which constitutional tissue was not available, only stop gain, splice site, probably damaging non-synonymous mutations or indels were considered as putative drivers. In order to minimize the chance of catching the germline variants, variants present in dbSNP137 which includes data from 1000 genomes ( www.1000genomes.org ) and Exome Variant Server ( http://evs.gs.washington.edu/EVS/ ) were excluded. Additionally, the variant was called a putative driver if it was reported in COSMIC v67 database, and/or if it was targeting one of the genes implicated in leukaemogenesis ( Supplementary Data 3 ). Candidate variants were validated by Sanger sequencing. Somatic copy number aberrations were retrieved from exome-sequencing data taking into account allelic coverage and percentage of reads for germline heterozygous variants. Sequence data can be accessed from http://seaseq.unige.ch/~nikolaev/raid_data1/ALLtotal_samples/ . CRLF2 analysis The PAR1 deletions were analysed in ALL samples, using 50 ng of genomic DNA, 1 U of amplitaq gold (Life Technologies, Paisley, UK), and primers C1423 and C1445, as described [13] . Thermal cycling conditions were 95 °C for 7 min and 30 s, followed by 35 cycles of 95 °C for 30 s, 66 °C for 30 s, 72 °C for 1 min and finally 1 × 72 °C for 9 min. The positive control primers were in the GATA1 locus; forward-5′-CGGAAGGATGGTATTCAGAC-3′, reverse-5′-TGTTACACACTCCACTCAGC-3′. Thermal cycling conditions were identical, except for annealing temperature; 57 °C. Statistical analysis Fisher exact one-sided test was used for mutual exclusion of the JAK–STAT and MAPK pathways. Somatic mutations from previously published 57 DS–AMKL samples were used in this study for evaluation of driver genes and pathways common between DS–ALL and DS–AMKL [16] , [18] . For this analysis, DS–AMKL samples were used, and for some comparisons also the advanced DS-TMD samples with driver mutations additional to GATA1. Accession codes: Exome sequence data for ALL samples from 39 DS patients have been deposited in GenBank/EMBL/DDBJ Sequence Read Archive under the accession code SRP044903 . How to cite this article: Nikolaev, S. I. et al. Frequent cases of RAS-mutated Down syndrome acute lymphoblastic leukaemia lack JAK2 mutations. Nat. Commun. 5:4654 doi: 10.1038/ncomms5654 (2014).